Heterogeneous stacking of nanodot monolayers by dry pick-and-place transfer and its applications in quantum dot light-emitting diodes Layered assembly structures composed of nanomaterials, such as nanocrystals, have attracted considerable attention as promising candidates for new functional devices whose optical, electromagnetic and electronic behaviours are determined by the spatial arrangement of component elements. However, difficulties in handling each constituent layer in a material-specific manner limit the 3D integration of disparate nanomaterials into the appropriate heterogeneous electronics. Here we report a pick-and-place transfer method that enables the transfer of large-area nanodot assemblies. This solvent-free transfer utilizes a lifting layer and allows for the reliable transfer of a quantum dot (QD) monolayer, enabling layer-by-layer design. With the controlled multistacking of different bandgap QD layers, we are able to probe the interlayer energy transfer among different QD monolayers. By controlling the emission spectrum through such designed monolayer stacking, we have achieved white emission with stable optoelectronic properties, the closest to pure white among the QD light-emitting diodes reported so far. Recent technological advances in the heterogeneous integration of various nanomaterials, including nanocrystals, into three-dimensional (3D) multilyer structures have allowed for effective methods of utilizing the unique electrical and optical properties of these nanomaterials in one confined layout. The integration of foreign inorganic materials with high precision, for example, has enabled new compound architectures and versatility in manufacturing new compound architectures for multifunctional electronic devices [1] , [2] . One of the easiest ways to fabricate such 3D structures is through the simple stacking of various two-dimensional monolayers of assembled nanomaterials. To this end, is it important not only to ensure the high structural quality of the two-dimensional monolayer but also to maintain such quality during the stacking process. Semiconductor colloidal quantum dots (QDs) are some of the most important and attractive nanomaterials owing to their tunable optical and electronic properties [3] , [4] , [5] , and considerable effort has been devoted to the synthesis of high-quality, defect-free QDs with a narrow size distribution (<5%; ref. 6 ). Owing to their interesting properties and capability in bandgap engineering, QDs have been employed in various applications, including biosensing, light-emitting diodes and photovoltaic devices [7] , [8] , [9] , [10] , [11] , [12] . Considering the limited thickness of the active layer in these QD devices and the importance of thin-film quality control, the precise device structure control capability via the multistacking of monolayers offers an effective way to improve device performances and multifunctionalize such devices. A dry pick-and-place transfer approach is particularly desirable for monolayer transfer. Reliable and uniform multistacking of QD monolayers has not yet been realized by solution-state assembly methods, such as the Langmuir–Blodgett technique [13] and those using linker molecules [14] or electrostatic charges [15] , [16] , [17] , [18] . For example, dense packing between QD layers is difficult using the electrostatic method because of the repulsion between the charges on the QD surface and polymer layer. Many issues in these wet assembly methods could be avoided by using the dry assembly approach. In this paper, we present a novel way to transfer printing by introducing a lifting polymer layer as an eliminable container for the entire nanodot monolayer, which allows for the complete lift-off of the nanodots during the transfer process. This lifting layer is easily dissolved in water immediately before printing. Using this new method, we were able to reliably transfer monolayers and thus achieve multilayer stacking via layer-by-layer transfer, which results in stacked nanodot monolayers and even heterogeneous vertical combination of monolayers composed of various nanoparticles. We applied this technique to the QD systems and were able to control the energy bandgap structure and energy transfer rate between the QD monolayers for optoelectronic devices, offering stable luminous efficiency. The strategies reported here contribute greatly to the enhancement of the performance of white light-emitting diodes (WLEDs), which use multistacked QD monolayers as an active layer through controlled energy transfer and energy-level alignment for balanced white-light emission. 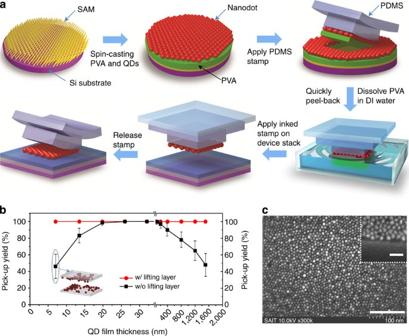Figure 1: Transfer printing of a nanodot monolayer. (a) Schematic illustration of the transfer-printing process for a nanodot monolayer. (b) QD pickup yield as a function of QD film thickness achieved by an elastomer stamp with a carrier layer (red circles) and without a carrier layer (black squares). The error bars are the s.d. in the pickup yields measured at a pressure of 196 kPa and a peeling rate of 80 mm s−1. Inset illustrates imperfect transfer of the QD monolayer of non-carrier layer case. (c) SEM image of the QD monolayer transferred by the process using a sacrificial layer. Scale bar, 100 nm. Inset shows a cross-sectional SEM image of the printed monolayer with 20° tilted angle (Scale bar, 20 nm). Nanodot monolayer transfer Figure 1a illustrates the steps of the nanodot monolayer transfer process using a water-soluble polymer as a lifting layer. We used polyvinylalcohol (PVA) whose molecular weight is ~10,000 Mw, to form a sacrificial layer that serves as a lifting layer. Before coating a donor substrate with PVA, the surface of the donor substrate was modified with covalently bound dense alkyl self-assembled octadecyltrichlorosilane (ODTS) monolayers to reduce the surface energy from 100 mJ m −2 (for hydrophilic Si) to 21 mJ m −2 (refs 19 , 20 ). The organic solvent of the QD solution, that is, cyclohexane, does not dissolve or swell PVA because cyclohexane is a nonpolar solvent, whereas PVA is a polar polymer. Therefore, QD monolayers are placed over the uniform PVA polymer layer by spin coating. As with the QDs on an ODTS self-assembled monolayer (SAM), a dense layer of QDs is formed on the top surface of the PVA layer by the interchain interactions associated with the van der Waals forces between the polymer chains and organic alkyl chain adhered to the nanocrystal surface [21] , [22] . There is a very weak interaction between the ordered alkyl chains of the ODTS monolayer and PVA, which allows QD/PVA layers from the donor substrates to be easily retrieved by kinetic control. Figure 1: Transfer printing of a nanodot monolayer. ( a ) Schematic illustration of the transfer-printing process for a nanodot monolayer. ( b ) QD pickup yield as a function of QD film thickness achieved by an elastomer stamp with a carrier layer (red circles) and without a carrier layer (black squares). The error bars are the s.d. in the pickup yields measured at a pressure of 196 kPa and a peeling rate of 80 mm s −1 . Inset illustrates imperfect transfer of the QD monolayer of non-carrier layer case. ( c ) SEM image of the QD monolayer transferred by the process using a sacrificial layer. Scale bar, 100 nm. Inset shows a cross-sectional SEM image of the printed monolayer with 20° tilted angle (Scale bar, 20 nm). Full size image Elastomeric polydimethylsiloxane (PDMS) stamps were laminated with donor substrates coated with QD/PVA. The low modulus of the PDMS stamp allows for good conformal contact between the stamp surface and QD monolayer over the entire area. After applying sufficient pressure, a fast retrieval of the stamp lifts the QD/PVA films off the handle silicon substrate. The adhesion between the QD layer and stamp is sensitive to the peeling rates owing to the viscoelastic behaviour of the elastomeric stamp [23] , [24] . The separation energy at the QD/stamp interface, G QD/stamp , depends strongly on the velocity of peeling according to the equation G QD/stamp = G PVA/ODTS-Si [1+ ø ( ν )], where ø is a function of the velocity ( ν ) and G PVA/ODTS-Si is the separation energy of the PVA–ODTS junction [24] , [25] . From this relation, the separation energy G QD/stamp ( ν ) is required to exceed G PVA/ODTS-Si . To achieve this condition, we applied a pressure of 196 kPa to the PDMS stamp and peeled the stamp back quickly at a peeling rate of 80 mm s −1 to successful transfer the QD/PVA layer. The measured dependence of the pickup yield on QD film thickness is shown in Fig. 1b . The pickup yield is defined as the ratio of the absorbance measured from the QDs before and after the pickup process. A relatively thick QD film (corresponding to a thickness of more than five to six layers) can be transferred by the conventional transfer-printing approach because binding between neighbouring QDs is sufficient to hold the entire film together as a single unit [26] . However, for a monolayer, insufficient coupling between the QDs results in the random transfer of isolated domains, which could potentially cause defects and short-current paths in the QD devices. Thus, it is essentially impossible to utilize the previous method for monolayer transfer. When picking up QDs without a lifting layer, the pickup yields of both the ultrathin layer and thick film (>300 nm) were very low, even with a sufficiently high peeling rate (>80 mm s −1 ). For a layer thickness of ~27 nm, the pickup yield achieved using a PDMS stamp reached 100% at an applied pressure of 196 kPa and a peeling rate of 80 mm s −1 . Such a complete transfer persists up to a thickness of 250 nm. The decreased pickup yields for thick films over 300 nm can be attributed to the spatial non-uniformity and poor surface roughness of QD assemblies because they were crudely prepared by drop casting, which involves solvent evaporation ( Supplementary Fig. S1 ). More densely ordered than such drop-casted thick QD films, ultrathin spin-coated films still exhibit low pickup yields owing to the lack of the aforementioned inter-QD coupling. In contrast to the previously discussed case, the QDs were all lifted up from the donor substrate during the pickup process using a lifting layer. As the SAM has the smallest interfacial free energy in the donor system, the separation occurred between the PVA and SAM layers. Thus, the carrier PVA layer was transferred to the PDMS stamp with the QDs. The polymer PVA with a tangled network structure was suitable for lifting isolated QDs regardless of the QD film thickness. The QD layers were successfully printed on receiver substrates after dissolving the PVA in deionized (DI) water. During this process, there was no damage by the solvents to the receiver substrates, such as the device stack, because the fully dried QD layers were transferred to the device stack after dissolving the PVA, as in a solvent-free process. The QD monolayers adhered to the PDMS stamps were successfully printed on silicon or glass substrates at a sufficiently low peeling rate (<0.1 mm s −1 ) because when printing QDs, the separation energy G QD/stamp ( ν ) should be lower than a threshold value, G QD/stamp crit ( ν )< G QD/receiver substrate crit (ref. 24 ). Scanning electron microscopy (SEM) images of the densely packed monolayer printed by the method described above are shown in Fig. 1c . As also shown in the tilted SEM image (inset, Fig. 1c ), the QD assembly printed on a silicon substrate is observed to be a monolayer without any vertically stacked QDs. A printed QD monolayer is clearly shown in a cross-sectional transmission electron microscopy (TEM) image ( Fig. 2a ). The QD monolayer was printed on a silicon substrate, followed by SiO 2 deposition by plasma-enhanced chemical vapour deposition to prepare the cross-section. An array of patterned QD monolayer stripes transfer-printed by a microstructured PDMS stamp is shown in the SEM images in Fig. 2b (see Supplementary Methods ). 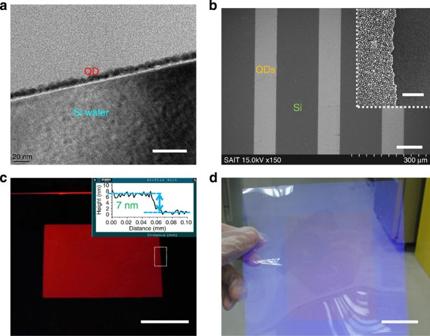Figure 2: Images of QD monolayers. (a) Cross-sectional TEM image of a QD monolayer on a Si substrate. Scale bar, 40 nm. (b) SEM image of patterned QD monolayer stripes transfer printed onto a Si substrate by the structured stamp. Scale bar, 100 μm. Inset shows magnified tilted SEM image of the edge of the patterned QD monolayer (Scale bar, 100 nm). (c) Optical fluorescence image of a QD monolayer printed on a glass substrate, excited by 365 nm ultraviolet irradiation. Scale bar, 2 cm. (Inset: the thickness measured from a surface profile of the right-side edge of the monolayer.) (d) Optical fluorescence image of a large-area QD monolayer printed on a flexible polyethylene naphthalate substrate, achieved by the repetitive lateral printing of monolayers. Scale bar, 4 cm. Figure 2c shows a fluorescence optical image of a QD monolayer printed on a glass substrate. The thickness of the QD monolayer was measured at several points over the entire area by a laser interferometer (NewView 7300 Zygo). The thickness measured along a surface profile of the right-side edge of the monolayer was 7 nm (inset, Fig. 2c ). A large-area transfer of monolayers could also be achieved on any flexible substrates by the repetitive lateral printing of monolayers. Figure 2d shows a photograph of an 8 × 10 cm monolayer transferred on a flexible polyethylene naphthalate substrate by four lateral printings under ultraviolet irradiation. The absorption intensity of the QD monolayer printed on a glass substrate corresponds to that of the spin-coated QD monolayer before transfer printing, suggesting no substantial loss during the entire transfer process ( Supplementary Fig. S2 ). By comparing the measured average absorption intensities before and after the transfer, the transfer yield was calculated to be 98.9±1.7% considering the error range of the instrument’s resolution ( Supplementary Note 1 ). Figure 2: Images of QD monolayers. ( a ) Cross-sectional TEM image of a QD monolayer on a Si substrate. Scale bar, 40 nm. ( b ) SEM image of patterned QD monolayer stripes transfer printed onto a Si substrate by the structured stamp. Scale bar, 100 μm. Inset shows magnified tilted SEM image of the edge of the patterned QD monolayer (Scale bar, 100 nm). ( c ) Optical fluorescence image of a QD monolayer printed on a glass substrate, excited by 365 nm ultraviolet irradiation. Scale bar, 2 cm. (Inset: the thickness measured from a surface profile of the right-side edge of the monolayer.) ( d ) Optical fluorescence image of a large-area QD monolayer printed on a flexible polyethylene naphthalate substrate, achieved by the repetitive lateral printing of monolayers. Scale bar, 4 cm. Full size image Multilayer stacking of nanodot monolayers We applied this transfer process to realize a heterogeneous multistacked structure. 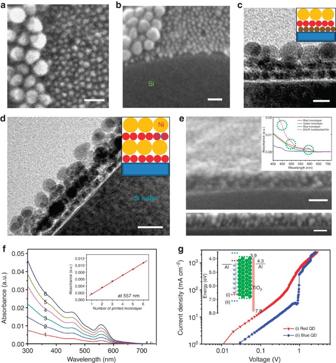Figure 3: Heterogeneous multistacking of nanodot monolayers. SEM images of the transfer-printed Ni nanoparticle monolayer on the printed QD monolayer. Top-view SEM images (a) and a tilted cross-sectional SEM image (b). Scale bar, 20 nm. Cross-sectional TEM images of the printed Ni/QD/Fe3O4monolayers (c) and of the alternatively printed Ni/QD/Ni/QD monolayers (d). Scale bar, 10 and 20 nm, respectively. (e) Tilted cross-sectional SEM image of a multistacked film composed of monolayers with different bandgap QDs. Scale bar, 20 nm. (Upper inset: absorbance of the red, green, blue and multistacked monolayers; lower inset: cross-sectional SEM image of a multistacked film after thermal annealing (scale bar, 20 nm)) (f) Absorbance of multistacked film composed of QD monolayers (inset: absorbance of the multistacked monolayers at 557 nm wavelength according to the number of printed monolayers). (g)J–Vcharacteristics of multistacked QD devices with a different bandgap QD monolayer next to the thick green QD layer (inset: energy band diagram of the device). Figure 3a,b shows SEM images of the transfer-printed monolayer of the nickel (Ni) nanodots encapsulated by aliphatic ligands on a QD monolayer printed on a Si wafer. The cross-sectional TEM images of the heterogeneous multistacked structures of nanodot monolayers composed of QD, Ni and iron oxide (Fe 3 O 4 ) nanoparticles in Fig. 3c,d show clear stacking of Ni/QD/Fe 3 O 4 monolayers and alternatively printed Ni/QD monolayers, respectively ( Supplementary Fig. S3 ). There is a large difference in the surface energies of the target substrates (100 mJ m −2 for hydrophilic Si, 1,140 mJ m −2 for clean Si in an ultra-high vacuum, 72 mJ m −2 for glass and 19.8 mJ m −2 for the PDMS) [20] , [27] , [28] , [29] . The surface energy of the QDs used in this work, which were encapsulated by aliphatic ligands, such as oleic acid, trioctyl amine and trioctyl phosphine, is 32.9 mJ m −2 , which guarantees the separation of the QDs from the PDMS stamps and printing them onto the QD layers owing to the low surface energy of the PDMS. Adhesiveless printing of the QD monolayers on another QD layer was facilitated by (i) heat-induced transfer with the assistance of shear force via thermal expansion of the PDMS or (ii) ligand exchange of the receiver QDs for increasing the surface energy of the receiver. To multistack the QD monolayers on the QD layer, the receiver substrate was annealed at 110 °C for 15 s after contacting the inked stamp with a receiver QD layer. Then, the stamp was slowly delaminated to print the QD monolayer. Printing a QD monolayer at a higher temperature for kinetically controlled transfer printing is advantageous because the critical energy release rate increases with increasing temperature [23] and the hydrophobic interaction associated with interchain-binding forces also increases [30] . In addition to the increased adhesion strength that is due to the high temperature, the shear force created by huge thermal expansion coefficient of the PDMS also promotes the transfer of the QD monolayers onto another QD layer by shear-enhanced transfer printing without adhesives [31] , [32] . The other alternative method is raising the surface energy of the printed QD monolayer (receiver) from 32.9 to 49.1 mJ m −2 through ligand exchange by crosslinking [12] . Both methods described above enabled stacking up to six layers, as shown in Fig. 3f , and in theory, there is no limit to in the number of QD layers that can be stacked. Figure 3: Heterogeneous multistacking of nanodot monolayers. SEM images of the transfer-printed Ni nanoparticle monolayer on the printed QD monolayer. Top-view SEM images ( a ) and a tilted cross-sectional SEM image ( b ). Scale bar, 20 nm. Cross-sectional TEM images of the printed Ni/QD/Fe 3 O 4 monolayers ( c ) and of the alternatively printed Ni/QD/Ni/QD monolayers ( d ). Scale bar, 10 and 20 nm, respectively. ( e ) Tilted cross-sectional SEM image of a multistacked film composed of monolayers with different bandgap QDs. Scale bar, 20 nm. (Upper inset: absorbance of the red, green, blue and multistacked monolayers; lower inset: cross-sectional SEM image of a multistacked film after thermal annealing (scale bar, 20 nm)) ( f ) Absorbance of multistacked film composed of QD monolayers (inset: absorbance of the multistacked monolayers at 557 nm wavelength according to the number of printed monolayers). ( g ) J – V characteristics of multistacked QD devices with a different bandgap QD monolayer next to the thick green QD layer (inset: energy band diagram of the device). Full size image Figure 3e shows a tilted SEM image of the multistacked heterogeneous film in the sequence of B/G/R QDs, achieved by performing three printing steps on a glass substrate. A green QD monolayer was printed on a blue QD monolayer, followed by the printing of a red QD monolayer on the green QDs. The absorbance of this multistacked film had three individual absorption peaks at wavelengths of 449, 509 and 591 nm, originating from each QD (upper inset, Fig. 3e ). The packing structure of the QD layers can be observed more clearly in the SEM image obtained after annealing (lower inset, Fig. 3e ). Figure 3f shows the absorbance of multistacked QD monolayers consisting of the same types of QDs. The peak absorption intensity at 557 nm increased linearly with an increasing number of monolayers, up to the sixth layer. The peak photoluminescence (PL) intensity as well as absorption intensity also increased linearly according to the number of printings of the monolayer ( Supplementary Fig. S4 ). The structural property of the obtained stacked multilayer in the in-plane and out-of-plane directions of the QD film was characterized by grazing incidence small-angle X-ray scattering results, and was compared with those of spin-coated and transfer-printed structures ( Supplementary Fig. S5 and Supplementary Note 2 ). We investigated the influence of QD monolayers with different bandgaps on the electron transport properties of the multistacked QD devices. Two different devices, one with a red QD monolayer located next to a thick green QD layer and the other with a blue QD monolayer (both sides are sandwiched between Al electrodes) were fabricated by transfer printing. The 10-nm-thick TiO 2 layer is a hole-blocking layer (inset, Fig. 3g ). Figure 3g shows the J – V curves of the two devices. The blue QD monolayer device had an energy barrier of 0.2 eV, whereas the red QD monolayer device possessed a cascaded structure with no energy barrier. The current density of the red device was significantly greater than that of the blue device. In contrast, the J – V curve of the blue device exhibited a sharp increase near 0.9 V, implying the initiation of electron tunnelling into the blue QDs. The electron mobilities of the red monolayer/green QD and blue monolayer/green QD devices were measured to be 3 × 10 −4 and 1.56 × 10 −4 cm 2 Vs −1 , respectively, by the space-charge-limited current method ( Supplementary Note 3 ). Our data suggest that the charge transport properties of multistacked QDs could be controlled through the designed energy band structure. 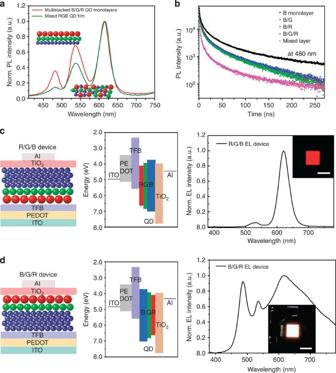Figure 4: Luminescence spectra from layered QD systems. (a) PL spectra of the multistacked QD monolayers and mixed QD layer. (b) Time-resolved PL decay profiles of the multistacked QD monolayers and mixed QD layer probed at 480 nm. (c) EL device with a multistacked QD layer in the sequence of R/G/B and its EL spectrum. Inset shows a photograph of EL emission from the device. Scale bar, 2 mm. (d) EL device with a multistacked QD layer in the sequence of B/G/R and its EL spectrum. Inset shows a photograph of EL emission from the device. Scale bar, 2 mm. Optoelectronic properties of QD-LEDs Figure 4a shows the normalized PL spectra of the sequentially stacked B/G/R QD monolayers as excitation at the 390 nm wavelength. The PL measured from a mixed QD layer with the same thickness (~19 nm) is also plotted for comparison. The individual PL emission from each QD can be clearly observed in both systems; however, the blue and green emission intensities were greatly suppressed in the mixed system. In our stacked monolayer system, energy transfer occurred mainly in the vertical direction (B→G and G→R) without considering energy transfer between the same bandgap QDs, whereas the energy transfer through the neighbouring interparticle interface occurred more frequently in all directions in the mixed system. Therefore, in the mixed system, energy transfer along the B→R QDs should also occur such that the PL intensity from the blue QDs is reduced considerably compared with that of the multistacked system, which suggests that the luminescence intensity at a specific wavelength can be selectively adjusted through controlled energy transfer by the sequence of multistacked monolayers. This relaxation dynamics of blue QDs is also shown in the results of the time-resolved PL measurements ( Fig. 4b ). We use a triple exponential decay model to fit the decay profile. The second fastest component, with a lifetime of ~10 ns, is considered for the analysis of Förster resonance energy transfer (FRET) of the QD films [14] . The decay was faster in the mixed layer system than that in the multistacked system, indicating that a relaxation process caused by FRET occurred. The increase in the probability of FRET caused the donor (mainly blue QD in this system) to undergo a further non-radiative decay process, whose rate increased with the relative concentration and distance of neighbouring QDs with smaller bandgaps. The PL decay time of the B/R film probed at a 480-nm wavelength was 8.8% faster than that of the B/G film. The PL decay time of the B/G/R film was 4.3% faster than that of the B/G film, suggesting a lower-energy transfer from the blue to red QDs in the B/G/R film. Figure 4: Luminescence spectra from layered QD systems. ( a ) PL spectra of the multistacked QD monolayers and mixed QD layer. ( b ) Time-resolved PL decay profiles of the multistacked QD monolayers and mixed QD layer probed at 480 nm. ( c ) EL device with a multistacked QD layer in the sequence of R/G/B and its EL spectrum. Inset shows a photograph of EL emission from the device. Scale bar, 2 mm. ( d ) EL device with a multistacked QD layer in the sequence of B/G/R and its EL spectrum. Inset shows a photograph of EL emission from the device. Scale bar, 2 mm. Full size image Our monolayer stacking was used to form active layers of LEDs. Control over the emission properties of these diodes was achieved by positioning QD layers of distinct sizes in various combinations. We used a structure composed of TFB and TiO 2 layers as hole- and electron-transporting layers, respectively. Figure 4c,d presents two different multilayer structures for WLEDs. The active layer of the first device consisted of one red monolayer, one green monolayer and four blue monolayers from the bottom to top (R/G/B device, Fig. 4c ). The second device had the reverse structure (B/G/R device, Fig. 4d ). The relative differences in the electroluminescent intensity of each QD were balanced by this combination while maintaining the optimum thickness of the active layer (~35 nm in our hybrid LED system). The exciton energy transfer from the higher- to lower-energy QDs was controlled by changing the sequence of the monolayers. The R/G/B device exhibited a dominantly red emission. (The green emission intensity was only 5.4% of the red emission intensity.) The recombination zone formed around red QDs because there was a large barrier between the hole transport layer (HTL) and QD layer. The electrons could easily reach red QDs because of the high electron mobility of the TiO 2 layer and the n -type behaviour of the CdSe-based QDs. In the B/G/R device shown in Fig. 4d , blue QDs were located in the same recombination zone near the HTL, but exciton energy transfer from the blue QDs to lower-energy QDs was possible. Therefore, the red and green QDs had a sufficient amount of energy for emission, and the measured emission spectrum indeed displayed similar amounts of red and blue emissions. The emission from the red QDs was combined with the broad emission from the surface midgap states of the blue QDs [33] , [34] , yielding broadband emission (450–780 nm) across most of the visible light spectrum. However, green emission from the B/G/R device was still lower than red and blue emissions, resulting in Commission Internationale de l’Eclairage coordinates of 0.41 and 0.40. This difficulty can be overcome by inserting a blue QD monolayer between the red and green layers, as shown in the schematic and TEM image in Fig. 5a (B/G/B/R device). The time-resolved PL data of Fig. 5b show the difference in PL decay time between the B/G/R and B/G/B/R devices probed at 540 nm. The decay time of the B/G/R was 21% faster than that of the B/G/B/R film owing to the existence of a non-radiative decay mechanism by the energy transfer (G→R). This finding indicates that the energy transfer from green to red was effectively prohibited and that green emission was enhanced in the B/G/B/R device such that emission much closer to pure white may be obtainable from the B/G/B/R device. 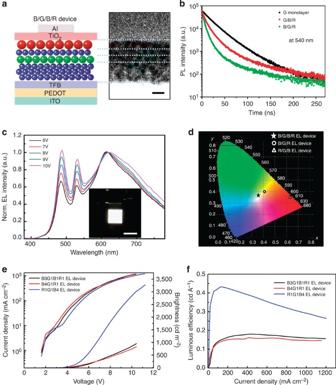Figure 5: Optoelectronic properties of QD WLEDs. (a) Cross-sectional TEM image of the EL device using a multistacked QD layer in the sequence of B/G/B/R and its schematic illustration. Scale bar, 10 nm. (b) Time-resolved PL decay profiles of multistacked films composed of B/G/B/R QD monolayers and B/G/R QD monolayers probed at 540 nm. (c) EL spectra of the B/G/B/R QD-LED according to the various applied biases. Inset shows a photograph of EL emission from the device. Scale bar, 2 mm. (d) Commission Internationale de l’Eclairage coordinates of light emission from the B/G/B/R, B/G/R and R/G/B QD-LEDs under a driving voltage of 10 V. (e)I–V–Lcharacteristics and (f) luminous efficiencies as a function of current density of the B/G/B/R, B/G/R and R/G/B QD-LEDs, respectively. Figure 5c shows the normalized electroluminescence (EL) spectra of a B/G/B/R device measured at various applied voltages. The spectra showed three main peaks at 488, 532 and 620 nm, which are ascribed to light emission from the blue, green and red QDs, respectively ( Supplementary Fig. S6 and Supplementary Note 4 ). The EL intensity of the signal from the green QDs was enhanced because the energy transfer from green to red decreased with the insertion of a blue QD monolayer between the green and red QD monolayers. Figure 5: Optoelectronic properties of QD WLEDs. ( a ) Cross-sectional TEM image of the EL device using a multistacked QD layer in the sequence of B/G/B/R and its schematic illustration. Scale bar, 10 nm. ( b ) Time-resolved PL decay profiles of multistacked films composed of B/G/B/R QD monolayers and B/G/R QD monolayers probed at 540 nm. ( c ) EL spectra of the B/G/B/R QD-LED according to the various applied biases. Inset shows a photograph of EL emission from the device. Scale bar, 2 mm. ( d ) Commission Internationale de l’Eclairage coordinates of light emission from the B/G/B/R, B/G/R and R/G/B QD-LEDs under a driving voltage of 10 V. ( e ) I – V – L characteristics and ( f ) luminous efficiencies as a function of current density of the B/G/B/R, B/G/R and R/G/B QD-LEDs, respectively. Full size image In Förster energy transfer, transfer efficiency ( E FRET ) can be obtained from the decay of time-resolved PL ( E FRET =1−( τ DA / τ D )), where τ DA and τ D are the decay lifetimes of a donor/acceptor (green/red) and donor (green) QD films, respectively. From the τ DA and τ D values in Fig. 4b , an E FRET (G→R) of 49% was obtained for the G/R QD layer ( Supplementary Fig. S7 and Supplementary Note 5 ). E FRET is also given by 1/(1+( R DA / R 0 ) [6] ), where the Förster radius ( R 0 , the distance where the energy transfer efficiency becomes 50%) can be calculated using the E FRET value and the donor–acceptor separation ( R DA ≈5.60 nm in Fig. 5a ). With the obtained Förster radius of 5.59 nm, the decrease in E FRET (G→R) in the G/B/R QD layer can be estimated using the known donor–acceptor separation distance of the G/B/R layer (10.9 nm). The resulting E FRET (G→R) was 1.8%, indicating that the non-radiative decay was reduced from 49 to 1.8% with the insertion of a blue QD monolayer as a spacer layer between the green and red QD layers. Therefore, the intensity of green EL emission in the B/G/B/R device increased to twice that of the B/G/R device. As a result, the Commission Internationale de l’Eclairage coordinates of this device observed under a driving voltage of 10 V were 0.36 and 0.37 ( Fig. 5d ). Figure 5e,f shows current density and luminance curves versus the applied bias for the R/G/B, B/G/R and B/G/B/R devices. The threshold voltage of the B/G/R and B/G/B/R devices were similar to that of the blue QD LED, and the peak brightness and luminance of the B/G/B/R device reached 1,040 cd m −2 and 0.19 cd A −1 , respectively, with balanced white-light emission. The peak brightness and luminous efficiency of the R/G/B device were higher (3,380 cd m −2 and 0.44 cd A −1 , respectively) than those of the other devices owing to the EL emission from the red QDs in the recombination zone. The emission from the red and green QDs in the B/G/R device was mainly because of the energy transfer from the blue QDs. It is noteworthy that the luminous efficiencies of the B/G/R and B/G/B/R devices exhibited better stability with an increase in the current density, whereas the R/G/B device exhibited a drop in efficiency. In the R/G/B device, there are an enormous number of excitons waiting for radiative recombination at large bias; thus, there is little room for the injected electrons and holes to form additional excitons. Additional electrons and holes simply pass through the device in this case. In contrast, in the B/G/R and B/G/B/R devices, excitons in the blue QD trilayer generate EL emission through radiative decay, and at the same time, part of excitons contributes energy transfer to the lower bandgap QDs of the upper layers, which leads to the faster decay time of the blue QDs, as discussed in Fig. 4b . Therefore, subsequently injected carriers can also recombine in blue QD layers, generating new excitons, and continuously contribute to energy transfer as well as EL emission even at a higher-magnitude electric field, which results in stable luminous efficiency against current density. The methodology described here offers the ability to transfer print and controllably stack large-area QD monolayers. Using this technique, the charge transport behaviour by energy band alignment and individual EL intensities from each QD associated with energy transfer were structurally controlled. A QD-LED, exhibiting light emission closer to pure white than the QD-WLEDs reported to date was obtained with stable operation as a result of integrating 3D multistacked systems into optoelectronic devices. These results might be useful for the heterogeneous integration of QD monolayers into other functional semiconducting films or other types of nanomaterials, as well as the multistacking of disparate QD monolayers. The use of these stacked assemblies on plastic substrates for flexible electronics and other unusually formatted electronics, as well as multilayer configurations with controlled energy band structures, could also be valuable. Materials CdSe/CdS/ZnS (core/shell/shell) QDs for the red-emissive QD, CdSeS/ZnS QDs for the green-emissive QDs and CdS/ZnS QDs for the blue-emissive QD were synthesized in the laboratory and used in this research. Ni nanoparticle (~15 nm) and Fe 3 O 4 nanoparticle (~7 nm) were also synthesized and used. The synthetic methods of the nanodots are described in Supplementary Methods . Donor substrate preparation ODTSs were treated on a ultraviolet–ozone-activated silicon substrate according to the method described by Kim et al. [26] These alkylsilane monolayers formed strong covalent bonds with the native oxide layer across the entire silicon substrate through Si-O-Si bonding. The covalently bonded ODTS-SAM was prepared with a high packing density and molecularly flat over a large area, with a surface roughness of ~0.2 nm, which resulted in a uniform and smooth PVA (Sigma-Aldrich) layer over a wide area through spin coating. PVA solution of 2 wt% dissolved in DI water with a molecular weight of 10,000 was filtered and spin coated at 1,500 r.p.m. for 60 s on the molecularly flat ODTS-treated Si substrate to form a 50-nm-thick sacrificial carrier layer. QDs dissolved in cyclohexane were spin coated on top of the PVA layer ( Supplementary Methods ). Transfer printing A slab of PDMS (Dow-Sylgard 184) was cast on a flat silicon wafer and cured at 75 °C in an oven for 2 h. Stamps with a thickness of 9 mm were laminated against donor substrates coated with QDs such that conformal contact was achieved, and the stamps were then quickly peeled back to lift off the QD/PVA films after applying sufficient pressure. The interfacial contact area between the QD film and stamp also influences the efficiency of the pickup process [25] . Sufficient pressure was applied to the stamp for full contact with QDs owing to the spherical shape of the QDs. The stamp inked with QDs/PVA was soaked in DI water for 1 h. After dissolving PVA layer, water droplets on the surface of the QD/stamp were removed by dry N 2 blowing. Stamps with only QD layers were brought into contact with receiver substrates, that is, glass, silicon, plastic substrates and ITO glasses precoated with a polymer HTL and HIL ( Supplementary Figs S8, S9 and Supplementary Note 6 ). Adhesiveless printing was facilitated by the large differences in the surface energies of the target substrates and the viscoelastic effects associated with the low peel-back rates of the stamps [29] . The transfer of QDs from the stamp to the HTL was accomplished more easily than the pickup process because the polymer film (HTL) served as a glue to forge a strong bond between the QDs and substrate [35] . For printing of a QD monolayer on receiver QD layers, heating of the receiver or control of the surface energy of the receiver QD layer were carried out. The pressures applied to the stamps and z axis-moving velocity were controlled by a custom-built automated machine consisting of motion-controlled X, Y, Z stages with 1 μm resolution and dual optical vision systems. Thickness measurement Thickness of QD monolayers were characterized by NewView 7300 Zygo. The optical instrument is a laser interferometry performed by scanning white-light interferometry technology providing fast, non-contact, high-precision 3D metrology of surface features with <1Å resolution in vertical direction. Contact angle measurement Contact angle measurements of various solvents on QD films were performed with a DSA 10-MK2 instrument using a drop shape analysis system. Approximately 10 μl of the solvents was dropped on QD films by a microsyringe, and the images of the droplet were obtained using a digital camera. The reference solvents used were ethylene glycol, diiodomethane and DI water for accuracy of the measurement. The surface energies of the receiver, including QD films and substrates, were calculated using Fowkes theory. QD PL lifetime measurements Using spectrally and time-resolved PL spectroscopy, we undertake energy transfer studies of stacked QD monolayer samples. Time-resolved PL decays were obtained by a time-correlated single-photon-counting module in Nanofinder 30 (Tokyo Instruments, Japan). Mixed or stacked QD samples on quartz substrates were excited at 405 nm with ~100 ps pulses and a repetition rate of 2.5 MHz from a pulsed diode laser (Picoquant PDL 800-B). The PL was spectrally dispersed in a monochromator (150 grooves per mm grating) with 12.75-nm spectral resolution and detected with a single-photon avalanche diode (PerkinElmer, SPCM-AQR-14-FC). The detection system was coupled to a photon-counting module (Becker & Hickl, PMS) with a 350-ps timing resolution. The pulsed laser and time-correlated single-photon-counting system provided a time window of 400 ns and an instrumental response function of 0.75 ns. Printed QD-LED fabrication and characterization Patterned ITO glass precoated with TFB and PEDOT was prepared, and red-, green- and blue-emitting QD monolayers were transfer printed on top of the printed QD layers or TFB layer. Crosslinking of the QDs and thermal annealing were performed according to a previously reported method [12] . A sol-gel TiO 2 layer acting as an electron transport layer (ETL) was spin coated at 2,000 r.p.m. for 30 s and then annealed at 100 °C for 15 min under ambient conditions. An aluminium electrode was thermally evaporated on top of the ETL as cathode under a high vacuum (10 −6 Torr), and thermal annealing after Al deposition was carried out at 140 °C for 20 min in a nitrogen atmosphere. Encapsulation was followed using cover glass in a nitrogen glove box. EL spectra, current density–voltage ( J – V ) and luminance–voltage ( L – V ) characteristics were recorded using a Spectrascan PR650 spectrophotometer coupled with a Keithley 238 voltage and current source measurement unit. All measurements were performed under ambient conditions. How to cite this article: Kim, T.-H. et al. Heterogeneous stacking of nanodot monolayers by dry pick-and-place transfer and its applications in quantum dot light-emitting diodes. Nat. Commun. 4:2637 doi: 10.1038/ncomms3637 (2013).